Experimental generation of an eight-photon Greenberger–Horne–Zeilinger state Multi-partite entangled states are important for developing studies of quantum networking and quantum computation. To date, the largest number of particles that have been successfully manipulated is 14 trapped ions. Yet in quantum information science, photons have particular advantages over other systems. In particular, they are more easily transportable qubits and are more robust against decoherence. Thus far, the largest number of photons to have been successfully manipulated in an experiment is six. Here we demonstrate, for the first time, an eight-photon Greenberger–Horne–Zeilinger state with a measured fidelity of 0.59±0.02, which proved the presence of genuine eight-partite entanglement. This is achieved by improving the photon detection efficiency to 25% with a 300-mW pump laser. With this state, we also demonstrate an eight-party quantum communication complexity scenario. This eight-photon entangled-state source may be useful in one-way quantum computation, quantum networks and other quantum information processing tasks. The creation and coherent manipulation of multi-photon entangled states has a crucial role in photonic quantum-information processing. In most cases, a pulse-pumped spontaneous parametric down-conversion (SPDC) process is used for the generation of multi-photon entangled states in which n photon pairs from the SPDC's n th-order emission are available. In particular, polarization-entangled Einstein–Podolsky–Rosen (EPR) pairs are often used as the basic blocks for generating multi-photon entangled states or as resources for performing quantum teleportation tasks. A number of experiments involving two photon pairs [1] , [2] , [3] , [4] , [5] , [6] , [7] , [8] and a few experiments involving five photons (two photon pairs plus one single photon) [9] or three photon pairs [10] , [11] , [12] , [13] have been carried out to demonstrate various protocols in quantum communication and linear optical quantum computing. Typical systems for two-photon-pair experiments use a frequency-doubled Ti:sapphire mode-locked laser as a pump, with a repetition rate of ~80 MHz, a pulse duration of ~150 fs, and an operating wavelength of ~400 nm. The improvement in moving from two-photon-pair to three-photon-pair experiments depends on the pump power being increased from 600 mW to 1 W through the use of a high-power continuous-wave laser to pump the mode-locked laser [14] . However, the sixfold coincidence count rates under this pump power are still low, and it is difficult to increase the pump power further in order to manipulate more photon pairs. In fact, other methods have been developed in recent years that are capable of generating more photon pairs under moderate pump power, such as sources obtained using spontaneous processes in waveguide structures [15] or photonic crystal fibres [16] , [17] . More recently, an ultraviolet enhancement cavity suitable for multi-photon experiments was implemented by Roland Krischek et al . [18] This system can provide greater than 7 W ultraviolet pump power for SPDC processes, which also makes the generation of more photon pairs possible. However, because of the nature of spontaneous processes, the probability μ of generating one photon pair per pump pulse should normally be restricted to less than 0.1 such that the noise from higher order photon-pair emission can be neglected. For an experiment involving n photon pairs from a spontaneous process, the 2 n -fold coincidence counting rate can be roughly estimated as C 2 n = fμ n η 2 n , where f is the pump laser repetition rate and η is the total detection efficiency, which is the product of all efficiencies between the source and detector. Thus, under the limit of μ ≤0.1, a key parameter for a good multi-photon source is the value of η , which significantly affects C 2 n , especially for large n . In this study, for the first time, we demonstrate an experiment involving genuine eight-photon entanglement, which is achieved by improving η to 0.25 and setting μ to be 0.046. With this source, we demonstrate an eight-party quantum communication complexity scenario using an eight-photon Greenberger–Horne–Zeilinger (GHZ) state with a fidelity of F =0.59±0.02. Our experimental result has a success probability largely exceeding the classical limit of 56.25%, which shows that the eight-photon entangled state we prepared violates the Mermin inequality [19] . Theoretical schemes Communication complexity problems (CCPs) [20] describe the communication cost incurred in performing distributed computation tasks among a number of separated parties, with each party holding his or her own input data at the beginning. As the quantum mechanical counterpart of CCPs, quantum communication complexity problems (QCCPs) involve the same problems, but the different parties communicate by sending quantum bits instead of classical bits [21] (or by sending classical bits through previously shared entanglements [22] ). It has been shown [23] , [24] that QCCPs can have quadratic or even exponential superiority over classical communication complexity in some cases. It has also been proven that a violation of Bell inequalities is the necessary and sufficient condition for QCCPs to outperform classical CCPs [25] . The special quantum communication complexity scenario (QCCS) that we demonstrate in our experiment is an eight-party version of Buhrman's model [26] . Suppose that there are eight parties A 1, A 2,..., A 8 receiving data X 1 , X 2 ,..., X 8 , respectively, where X i U {0, 1} 2 , i =1, 2,...,8, and The common objective of each party is to obtain the correct value of the Boolean function X 1 ,..., X 8 can each be written in binary notation as x 1 1 x 1 0 ,..., x 8 1 x 8 0 . Under the conditions of equation (1), for any input X 1 ,..., X 8 , the value distributions of x 1 0 ,..., x 8 0 should be one of 128 possible combinations, which can be divided into five groups, namely, 0 8 , 0 6 1 2 , 0 4 1 4 , 0 2 1 6 and 1 8 . Here 0 i 1 j stands for a combination that has i bits of 0 and j bits of 1, regardless of the order in which they appear. The Boolean function F can be rewritten as where That is, F 0 =0 for the groups 0 8 , 0 4 1 4 and 1 8 , whereas F 0 =1 for 0 6 1 2 and 0 2 1 6 . In the classical situation, the maximum success probability for this scenario is where N is the number of parties. In our case, N =8 so that . Using quantum protocols, the eight parties X 1 − X 8 that share a prior eight-qubit GHZ state can have a success probability of . The protocol is shown below. The eight-qubit GHZ state is Each party holds a qubit of and applies rotations R ( x ) or R ( y ) to the qubit according to the value (that is, 0 or 1) of its own classical bit xi 0 , i ∈ 1, 2...8, where Next, the party measures its qubit in the 0/1 basis and obtains the result yi ∈ {0, 1}. After that, each party X i broadcasts a bit and can derive the correct value of F as with a success probability of 100%. Experimental realization of eight-photon GHZ state and QCCS We now proceed with the experimental description of how to generate the eight-photon GHZ state and demonstrate the QCCS scheme. Four specially designed ultrabright 'beam-like' EPR sources (S1 to S4) [27] were used in the experiment to provide polarization-entangled EPR photon pairs. 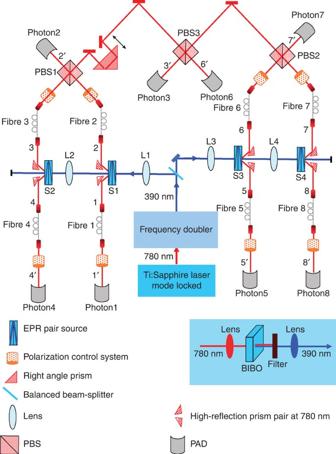Figure 1: Experimental set-up for generating the eight-photon GHZ state and demonstrating eight-party QCCS. A light pulse from a mode-locked Ti-sapphire laser with a duration of 140 fs, a repetition rate of 76 MHz, and a central wavelength of 780 nm first passes through a frequency doubler. The ultraviolet pulse with a power of 600 mW from the doubler is split into two beams by a balanced beam-splitter and is focused onto four pairs of BBO crystals to provide four EPR photon pairs. A collaborating and focusing system composed of four lenses is used to place beam waists of ~90 um exactly at the four EPR pair sources (S1–S4, containing a pair of beam-like-type cutting BBO crystals) to achieve high brightness. Down-converted photons are coupled into single-mode fibres at a distance of 25 cm from the EPR pair source. A polarization control system composed of two HWPs and one tiltable QWP is used for each single-mode fibre to correct the polarization variation caused by the fibre. A lens with a focusing length of 75 mm is placed before each single-photon detector to couple the output of single photons from the fibres. Each photon is measured with a polarization analysing detector (PAD), which is composed of a HWP, a QWP, an interference filter with a FWHM of 3 nm, a PBS, and two single-photon detectors. All 16 single-photon detectors had quantum efficiencies higher than 65% at 780 nm. The inset shows the set-up of the frequency doubler. In the frequency doubler, the 780-nm laser beam from the Ti:Sapphire laser was focused onto a 8 mm × 8 mm × 1.5 mm BiB3O6 (BIBO) crystal with af=125 mm lens. A high-performance short-pass filter was placed after the BIBO to clean up the residual red light from the outputted 390 nm laser beam. Finally, af=50 mm lens was used to collimate the 390 nm laser beam. The experimental set-up is illustrated in Figure 1 . A pulsed ultraviolet laser beam was split into two beams by a 50/50 nonpolarizing beam-splitter, and each beam was subsequently passed through two pairs of β-barium borate (BBO) crystals serving as the pump. Finally, 4 EPR pairs were generated in 8 different spatial modes, numbered from 1 to 8. The reason for using two pump beams, each generating two EPR pairs, instead of using one pump beam generating four EPR pairs, was to reduce the number of lenses that the pump beam passed through before pumping the latter two EPR sources (S3 and S4). Passing through too many lenses would lead to a large decrease in the down-converted photon detection efficiency, for example, a decrease from 0.23 to 0.21. Furthermore, all of the lenses were optimized according to their focal lengths to obtain the highest collection efficiency η and a moderate production efficiency μ . The focal lengths of L1, L2, L3 and L4 were 150 mm, 85 mm, 150 mm, and 85 mm, respectively, and the distances between S1 and S2 and between S3 and S4 were both 300 mm. Figure 1: Experimental set-up for generating the eight-photon GHZ state and demonstrating eight-party QCCS. A light pulse from a mode-locked Ti-sapphire laser with a duration of 140 fs, a repetition rate of 76 MHz, and a central wavelength of 780 nm first passes through a frequency doubler. The ultraviolet pulse with a power of 600 mW from the doubler is split into two beams by a balanced beam-splitter and is focused onto four pairs of BBO crystals to provide four EPR photon pairs. A collaborating and focusing system composed of four lenses is used to place beam waists of ~90 um exactly at the four EPR pair sources (S1–S4, containing a pair of beam-like-type cutting BBO crystals) to achieve high brightness. Down-converted photons are coupled into single-mode fibres at a distance of 25 cm from the EPR pair source. A polarization control system composed of two HWPs and one tiltable QWP is used for each single-mode fibre to correct the polarization variation caused by the fibre. A lens with a focusing length of 75 mm is placed before each single-photon detector to couple the output of single photons from the fibres. Each photon is measured with a polarization analysing detector (PAD), which is composed of a HWP, a QWP, an interference filter with a FWHM of 3 nm, a PBS, and two single-photon detectors. All 16 single-photon detectors had quantum efficiencies higher than 65% at 780 nm. The inset shows the set-up of the frequency doubler. In the frequency doubler, the 780-nm laser beam from the Ti:Sapphire laser was focused onto a 8 mm × 8 mm × 1.5 mm BiB3O6 (BIBO) crystal with a f =125 mm lens. A high-performance short-pass filter was placed after the BIBO to clean up the residual red light from the outputted 390 nm laser beam. Finally, a f =50 mm lens was used to collimate the 390 nm laser beam. Full size image To achieve the best stability of the system, eight polarization-preserving single-mode fibres were placed as close as possible to the BBO crystals to collect the down-converted photons in the eight spatial modes. In addition, we also constructed a new type of frequency doubler to improve the total detection efficiency η (Methods), which significantly increases the eight-photon coincidence rate without increasing the generation probability μ , thus keeping the noise of higher order photon-pair-emission from increasing. With these techniques and using only 300 mW pump power for each 'beam-like' EPR source, we observed ~22×10 4 s −1 photon pairs from each EPR source. The photon pairs were prepared according to the Bell state , where H and V denote horizontal and vertical polarization, respectively. The visibility with respect to the H / V (+/−) basis under 300 mW pump power was measured to be 96% (93%) where . The outputs of these fibres were directed to polarization beam-splitters (PBS) to perform post-selected fusion operations [28] between modes 1 and 3 (PBS1), and 6 and 7 (PBS2) or polarization-projection measurements for modes 1, 4, 5 and 8. Next, the transmitted modes of mode 3 and 7 after PBS1 and PBS2 were directed to PBS3 for another fusion operation. An eight-photon GHZ state was prepared by postselecting one and only one photon in each of the eight modes labelled 1′, 2′, 3′, 4′, 5′, 6′, 7′ and 8′. Next, in each mode, a quarter wave-plate (QWP) and half-wave-plate (HWP) were used to perform the R ( x ) or R ( y ) rotations (depending on the value of xi 0 ), and a PBS was placed after the HWP to derive the H / V basis measurement, where a result of | H › denotes 0 and a result of | V › denotes 1. Finally, the photons were spectrally filtered (Δ λ FWHM =3 nm) for good temporal indistinguishability and detected by space-coupled single-photon detectors for better collection efficiency. Note that the spatial modes were filtered by previous single mode fibres. Two single-photon detectors were employed for each photon, with one to detect H polarization and the other to detect V polarization. A homemade, programmable, 16-channel coincidence unit was used to simultaneously register all possible coincidences among the 16 single-photon detectors. Because of the long data collection period in our experiment (~60 h for one measurement basis) and strong focus of the ultraviolet laser beam on down-conversion BBO crystals, we also proposed an anti-burning method to avoid damage to the BBO crystals caused by the laser beam. For this method, each EPR pair source was mounted on a translation stage that moved up and down repeatedly in a small region to reduce heating due to the strongly focused ultraviolet pulses. This anti-burning system provided good stability to the pump power after it passed through the BBO crystals. Using this method, the stable time of the pump power (defined as the variation of pump power being less than ±2%) greatly increased from less than 2 h to months. It is also worth noting that in our experiment, the interference of two independent photons occurred between the outputs of two single-mode fibres mounted on stable translational stages. This adaptation greatly improved the stability of our interferometer. Under 300 mW pump power for each SPDC source, the average visibility of Hong–Ou–Mandel (HOM) interferences between independent photons overlapped on PBS1, PBS2 and PBS3 was observed to be ~73%. 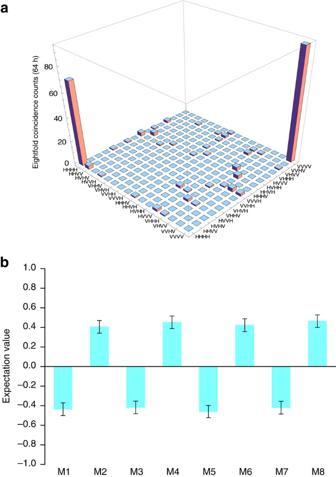Figure 2: Entanglement witness measurement results of eight-photon GHZ state. (a) Eightfold coincidence counts measured inH/Vbasis over 64 h. The sum of all 256 columns was 219, while the sum of the two desired columnsHHHHHHHHandVVVVVVVVwas 165. (b) Measured expectation values ofMk,k=1,...,8. The data collection time of eight-photon coincidence counts for eachMkwas ~48 h. The sum of all 256 kinds of eight-photon coincidence counts for eachMkwas ~195. The error bars correspond to the counting statistics. We can verify genuine eight-photon entanglement of our prepared eight-photon GHZ state using the witness [29] where and The state fidelity can then be directly calculated as Figure 2a shows the eightfold coincidence counts of our prepared eight-photon GHZ state measured in H / V basis. Approximately 80 eight-photon events were observed in 64 h for the two desired columns of HHHHHHHH and VVVVVVVV , while undesired events in the other 254 columns clearly showed effects from the higher order photon-pair emissions in our experiments. The effect from PBS imperfections was small, because every PBS in our system had an extinction ratio of more than 300:1 for both output ports. From Figure 2a , the value of observable was calculated to be 0.75±0.03. Figure 2b illustrates the expectation values of M k , k =1, ..., 8. Each expectation value was derived from a complete set of eight-photon coincidence counts (256 kinds) obtained by measuring each photon on the basis of . We obtained an averaged expectation value of (−1) k M k of from Figure 2b . Therefore, we can evaluate the expectation value of W G as ‹ W G ›=−0.09±0.02, which clearly shows the presence of genuine eight-photon entanglement. Therefore, the fidelity of our prepared GHZ state was according to equation (11). Figure 2: Entanglement witness measurement results of eight-photon GHZ state. ( a ) Eightfold coincidence counts measured in H / V basis over 64 h. The sum of all 256 columns was 219, while the sum of the two desired columns HHHHHHHH and VVVVVVVV was 165. ( b ) Measured expectation values of M k , k =1,...,8. The data collection time of eight-photon coincidence counts for each M k was ~48 h. The sum of all 256 kinds of eight-photon coincidence counts for each M k was ~195. The error bars correspond to the counting statistics. Full size image To demonstrate the eight-party QCCS, there were 128 kinds of possible inputs of X 1 , ..., X 8 , and eight communication parties were expected to perform different local rotations on their qubits for different inputs. Measuring all 128 possible cases was difficult, because of the long data-collection period of ~50 h for each case. The 128 possible cases were thus divided into five groups denoted 0 8 , 0 6 1 2 , 0 4 1 4 , 0 2 1 6 and 1 8 , as mentioned above. Therefore, in our experiment, we only studied one case in each group (that is, 00000000, 11000000, 11110000, 11111100, and 11111111). Because of the symmetry of our state-generation setup, it is reasonable to assume that exchanging the places of 1 and 0 among the eight parties would yield no differences in the experimental results. 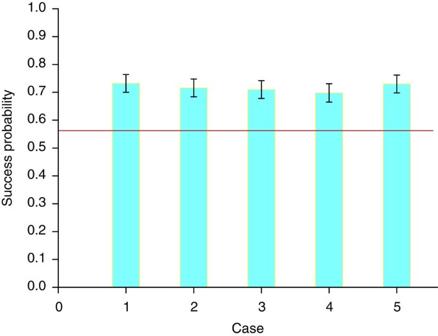Figure 3: Experimental QCCS success probabilities for five cases. Cases 1 to 5 denote groups 08, 0612, 0414, 0216and 18, respectively. The solid red line shows the classical limit of 56.25%. The error bars correspond to the counting statistics. Figure 3 shows the measured success and fail probabilities of the five cases. In each group, the success probability P s largely exceeded the classical limit of 56.25%. In addition, the average success probability Pa was 71.7±1.4%. In other words, the eight-photon state we prepared cannot be described by local realistic theory. Figure 3: Experimental QCCS success probabilities for five cases. Cases 1 to 5 denote groups 0 8 , 0 6 1 2 , 0 4 1 4 , 0 2 1 6 and 1 8 , respectively. The solid red line shows the classical limit of 56.25%. The error bars correspond to the counting statistics. Full size image The imperfections in our experiment had two main causes. One cause involved the distinguishability between two independent photons and an imperfect EPR source, which were characterized by the HOM interference visibility V HOM of independent photons and the entanglement visibility V Ent of the EPR source measured under low pump power. In our experiment, V HOM and V Ent were ~82% and 97%, respectively. The other important factor was the higher order photon-pair emissions due to the nature of SPDC processes. The effect of this factor can be directly observed from the 256 measured eight-photon counts in the H / V basis. In summary, we have presented a novel source that can provide four independent EPR photon pairs for multi-photon experiments using only 300 mW pump power for each SPDC source. The experimental setup of this source is rather simple, stable and easy to manipulate. Using four EPR photon pairs and three fusion operations, we successfully generated an eight-photon GHZ state with verified genuine eight-photon entanglement. With this GHZ state, we demonstrated an eight-party quantum communication complexity scenario in an experiment, with the result exceeding the classical limit of the eight-party communication complexity scenario. A number of further applications can be imagined with our eight-photon entanglement source; for instance, the demonstration of various protocols in multiparty quantum networking [12] , [30] , loss-tolerant one-way quantum computing using cluster states [31] , high-resolution quantum optical metrology with multiphoton states [32] , and tests of Bell's theorem without inequalities and alignments [33] . In recent years, the planar integrated optics approach of optical quantum circuits has shown tremendous potential for future optical quantum information processing, such as Shor's algorithm being demonstrated on a chip with four single photons [34] . The integrated optics approach has the advantages of perfect spatial overlap and a compact and stable set-up compared with traditional table-optics systems. Therefore, the possible combination of our high-brightness, high-collection-efficiency SPDC source and planar integrated optics might bring further advancement to optical quantum information technology in the future. Frequency doubler for high photon-collection efficiency The collection efficiency of the photon pairs from the SPDC source was an important factor in reducing the data collection time in our eight-photon experiment. On the basis of our previous beamlike EPR source [27] , we created a new type of frequency doubler that remarkably improved the photon-pair collection efficiency. The experimental set-up of our frequency doubler is shown in the inset of Figure 1 . In our frequency doubler, we used a BiB 3 O 6 (BIBO) crystal instead of a LiB 3 O 5 (LBO) or BBO crystal, and the BIBO crystal was cut at θ =149.5° and φ =90° to perform a type I second-harmonic generation (SHG) process. We found that the spectral bandwidth of the output ultraviolet beam from our frequency doubler was narrower than other frequency doublers that use LBO or BBO crystals. In our case, the spectral bandwidth of the 390 nm laser beam was 0.9 nm (full width of half-maximum (FWHM)). Such a narrow bandwidth of pump significantly improves the down-converted photon-pair collection efficiency. We also found that to achieve the best collection efficiency of photon pairs, the value of the BIBO's phase-matching angle θ should be slightly different from the value of the highest SHG output power. Another improvement of the collection efficiency was achieved by ensuring that the focusing in the frequency doubler was not too strong. We chose a focal length of 125 mm for the focusing lens before the BIBO crystal to obtain the best collection efficiency while maintaining enough SHG output power. With the above-mentioned techniques and other arrangements for improving photon detection efficiency described in the main text, such as splitting the 390-nm pump beam into two beams and choosing optimized focal lengths for pump-beam focusing, we improved the average total detection efficiency η from the original value of 0.125 to 0.250. This result increased the eight-photon coincidence counting rate by over 200 times under the same generation probability μ , thereby making the eight-photon entanglement experiment feasible. It is important to note that because of the narrower spectral bandwidth of the 390-nm laser beam, the visibility of HOM interference between independent photons in our system decreased. In fact, when using the low power of a 390-nm laser beam (~50 mW) to remove the emission background of the higher order photon pairs, we observed an average HOM interference visibility of ~83% and ~90% when BIBO and BBO crystals were used in the frequency doubler, respectively. How to cite this article: Huang, Y.-F. et al . Experimental generation of an eight-photon Greenberger–Horne–Zeilinger state. Nat. Commun. 2:546 doi: 10.1038/ncomms1556 (2011).